A common functional promoter variant linksCNR1gene expression to HDL cholesterol level Type 1 cannabinoid receptor blockers increase high-density lipoprotein cholesterol levels. Although genetic variation in the type 1 cannabinoid receptor—encoded by the CNR1 gene—is known to influence high-density lipoprotein cholesterol level as well, human studies conducted to date have been limited to genetic markers such as haplotype-tagging single nucleotide polymorphisms. Here we identify rs806371 in the CNR1 promoter as the causal variant. We re-sequence the CNR1 gene and genotype all variants in a DNA biobank linked to comprehensive electronic medical records. By testing each variant for association with high-density lipoprotein cholesterol level in a clinical practice-based setting, we localize a putative functional allele to a 100-bp window in the 5′-flanking region. Assessment of variants in this window for functional impact on electrophoretic mobility shift assay identifies rs806371 as a novel regulatory binding element. Reporter gene assays confirm that rs806371 reduces gene expression, thereby linking CNR1 gene variation to high-density lipoprotein cholesterol level in humans. Clinical lipid disorders have enormous public health significance and increasing societal burden in developed countries [1] . High-density lipoprotein cholesterol (HDL-C) levels are inversely correlated with cardiovascular disease, and each 1 mg dl −1 decrease in HDL-C is associated with a 6% increase in adverse clinical events [2] . As HDL-C levels are highly heritable (H 2 ranging from ~0.4–0.7), there is great interest in characterizing the genetic architecture underlying this important complex trait [3] , [4] , [5] , [6] , [7] , [8] . The type 1 cannabinoid receptor (CB 1 ) is a novel therapeutic target for controlling lipoprotein metabolism. As CB 1 receptors within the brain influence eating behavior, rimonabant, a selective CB 1 antagonist, was initially designed to correct weight gain [9] , [10] . However, in large clinical trials, rimonabant improved HDL-C levels far greater than originally anticipated [9] , [10] , [11] , [12] . Likewise, variation in the CNR1 gene, which transcribes the CB 1 receptor, has previously been associated with HDL-C levels in several independent study cohorts [13] , [14] , [15] . We have previously reported that a common CNR1 haplotype (H4, frequency ~15% in the general population) is associated with decreased HDL-C levels, independent of body mass index (BMI) [13] . Interestingly, common non-synonymous single nucleotide polymorphisms (SNPs) have not been observed within the CNR1 coding region, and all studies assessing the impact of CNR1 gene variation on clinically recognizable traits have been conducted using ‘markers’ (haplotype-tagging SNPs). Therefore, the causal allele has not been identified. As such, we present here a series of polymorphisms in the CNR1 gene identified through deep re-sequencing, and we re-genotype these variants testing them for association with HDL-C levels in vivo , using the largest clinical practice-based DNA biobank in the United States [16] , [17] . Variants associated with HDL-C level were then further characterized experimentally in vitro , using electrophoretic mobility shift assays (EMSA) and gene promoter reporter (luciferase) assays. We now report that rs806371 is the likely causal variant linking CNR1 gene expression to HDL-C level. Identification of putative functional variants BioVU is a clinical practice-based biobank linked to comprehensive electronic medical records (EMRs) [17] . The largest resource of its kind ( n =157,719 on 10 January 2013), BioVU is robust in its ability to replicate genetic associations previously identified in disease-based cohorts [16] . Our previous analysis identified a CNR1 haplotype associated with HDL-C levels in extended families of Northern European ancestry [13] . To assess this relationship within the community, we sampled 1% of 100,000 BioVU subject records claiming European Ancestry for further study (50% female and 50% male subjects). The precision of ancestry data within BioVU has previously been validated using a panel of 360 ancestry informative markers [18] . 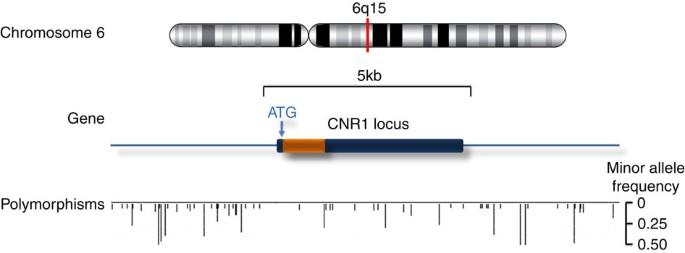Figure 1: Location of polymorphisms identified from re-sequencing. The figure illustrates chromosome location of theCNR1gene (upper panel), the region of re-sequencing (middle panel), and the locations as well as minor allele frequencies of all polymorphisms (lower panel). Clinical characteristics of the current BioVU sub-sample are shown in Table 1 . Table 1 Demographic characteristics of BioVU study cohort. Full size table To quantify variability across our locus of interest, the entire CNR1 gene (15 kb of genomic DNA) was re-sequenced in 95 individuals selected from the Utah Centre d’Etude du Polymorphisme Humain (CEPH) reference panel within HapMap (Coriell Cell Repository) ( Fig. 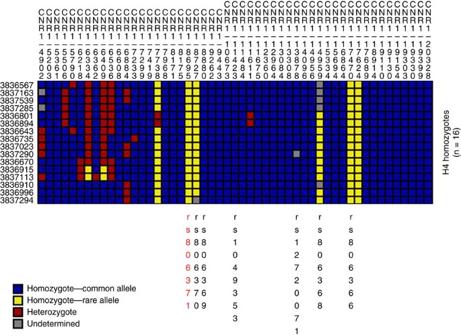Figure 2: Individual CNR1 genotypes display visually for all H4 homozygotes. The figure illustrates individual genotypes of all H4 homozygotes in the BioVU study cohort. The figure was generated using publically available data on Genome Variation Server 134 (http://gvs.gs.washington.edu/GVS134/). 1 , Table 2 ). A total of 65 polymorphisms were identified, including 62 SNPs and 3 insertion/deletions. Thirty-seven of these polymorphisms had not been reported previously (that is, did not have existing rsNumbers). All observed variants were re-genotyped in the BioVU sub-cohort from Table 1 ( n =1,006) using our high-throughput Sequenom platform (see Methods). As described in our previous study using clinical data derived from EMRs [19] , the primary endpoint in the BioVU sub-cohort was median outpatient HDL-C levels, adjusted for age and gender [14] . Other important clinical covariates were either extracted directly from the EMRs (for example, BMI nearest to the date on which each median HDL-C level was extracted) or defined using time stamps through natural language processing (for example, exposure to medications known to alter HDL-C levels) [20] . Figure 1: Location of polymorphisms identified from re-sequencing. The figure illustrates chromosome location of the CNR1 gene (upper panel), the region of re-sequencing (middle panel), and the locations as well as minor allele frequencies of all polymorphisms (lower panel). Full size image Table 2 CNR1 single SNP associations with HDL-C in the BioVU study cohort. Full size table Median HDL-C levels were then tested for association with each variant genotyped across the CNR1 locus ( Table 2 ). Using this strategy, we found three common CNR1 variants to be nominally associated with HDL-C level ( P <0.05, additive model): two in the 5′-flanking region (5′-FR) and one located in the 3′-untranslated region (3′-UTR). Both variants in the 5′-FR remained significant after adjustment for BMI ( Table 2 ): CNR1-8727 (dbSNP designation rs806370) and CNR1-8695 (dbSNP designation rs806371). None of the synonymous variants in the CNR1 coding region were found to be associated with HDL-C level. Although rare, two additional CNR1 variants were associated with HDL-C level after adjustment for BMI ( Table 2 ): (CNR1-11675 and CNR1-19154). These rare 3′ variants were tightly linked in our pair-wise allelic association analyses ( r 2 =1.0). However, due to their extremely low minor allele frequencies (2 alleles in 1,006 study subjects), these variants were not pursued further in our comparison with prior CNR1 risk haplotypes, or in our functional assessment of CNR1 gene expression in vitro . rs806371 is associated with HDL-C levels We have previously reported a common CNR1 haplotype associated with HDL-C level in families of Northern European ancestry [13] . 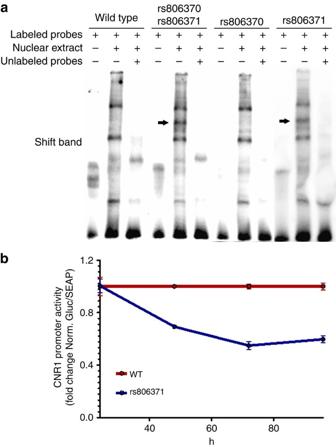Figure 3: rs806371 is a functional variant in theCNR1promoter. (a) The figures illustrate DNA-protein binding patterns analyzed by EMSA. Biotin-labeled double-stranded probes were incubated with nuclear extract from HEK293 cells. (Left) A diplotype probe carrying both rs806370 and rs806371 was compared with wild-type (WT) probe. (Right) DNA–protein binding patterns were compared between WT probe, and single variant probes carrying only rs806370 or rs806371. The additional shift bands are indicated by arrows. (b) The figure illustrates normalized fold change forCNR1promoter activityin vitro. Reporter gene constructs, with or without rs806371, were transient transfected into Huh-7 cells. Luciferase activities were measured at 48 72 and 96 h. Results represent mean±s.e. for experiments run in triplicate. As our re-genotyping of the CNR1 locus was comprehensive in the current study, we were able to reconstruct the previously reported risk haplotype, H4, in this BioVU sub-sample ( Table 3 ) [13] , [14] , [15] . Strikingly, the effect size and level of significance for association with HDL-C was identical for the H4 risk haplotype and for rs806371, our putative functional variant harbored within the 5′-FR. (HDL-C mean±s.d. was 53.47±16.30, 50.85±16.76 and 48.03±12.52 mg dl −1 for carriers of 0, 1 and 2 copies of the H4 risk haplotype; and HDL-C mean±s.d. was 53.47±16.45, 51.13±16.64 and 48.23±12.60 mg dl −1 for subjects with 0, 1 and 2 copies of the minor allele at rs806371.) Table 3 Effect size for HDL-C (mg dl −1 ) based on haplotypes reconstructed using tag SNPs from our prior work in families [13] . Full size table We therefore conditioned our findings for rs806371 and HDL-C on the tagging SNPs used previously to define the H4 risk haplotype. When we conditioned our findings for rs806371 on genotype at the adjacent variant rs806370, the significance of this relationship was attenuated (from P =0.026 to P =0.90, additive model), implying that the association was not solely driven by rs806371. Furthermore, when we did the converse (conditioned the analyses for rs806370 on rs806371), the association of HDL-C with rs806370 was also attenuated (from P =0.017 to P =0.54, additive model). As these observations suggest that both variants may contribute to the association, we screened all 5′ variants to quantify the strength of their linkage disequilibrium with the H4 haplotype using Genome Variation Server 134 at Seattle SNPs ( http://gvs.gs.washington.edu/GVS134/ ) ( Fig. 2 ), and we subsequently tested rs806370 and rs806371 for binding interactions with nuclear proteins using EMSA ( Fig. 3 ). Figure 2: Individual CNR1 genotypes display visually for all H4 homozygotes. The figure illustrates individual genotypes of all H4 homozygotes in the BioVU study cohort. The figure was generated using publically available data on Genome Variation Server 134 (http://gvs.gs.washington.edu/GVS134/). Full size image Figure 3: rs806371 is a functional variant in the CNR1 promoter. ( a ) The figures illustrate DNA-protein binding patterns analyzed by EMSA. Biotin-labeled double-stranded probes were incubated with nuclear extract from HEK293 cells. (Left) A diplotype probe carrying both rs806370 and rs806371 was compared with wild-type (WT) probe. (Right) DNA–protein binding patterns were compared between WT probe, and single variant probes carrying only rs806370 or rs806371. The additional shift bands are indicated by arrows. ( b ) The figure illustrates normalized fold change for CNR1 promoter activity in vitro . Reporter gene constructs, with or without rs806371, were transient transfected into Huh-7 cells. Luciferase activities were measured at 48 72 and 96 h. Results represent mean±s.e. for experiments run in triplicate. Full size image To begin assessing the causality of rs806371, we plotted genotypes for each CNR1 SNP in all 16 individuals currently found to be homozygous for the H4 haplotype described in our prior work ( Fig. 2 ); in this analysis, rs806371 was found to only occur on the H4 background. Although CNR1-7738, another CNR1 5′-FR variant, was also found to have increased prevalence on the H4 background ( Fig. 2 ), this variant was frequently present on other haplotypes (not shown), and its correlation with H4 was not robust ( r 2 =0.139). As such, we did not pursue CNR1-7738 in our subsequent functional studies. rs806371 creates a new regulatory element for CNR1 Electrophoretic mobility shift assays (EMSA) were then conducted to determine if nucleotide substitutions disrupt or induce any regulatory elements in the CNR1 promoter ( Fig. 3 ). As noted, rs806370 and rs806371 in the 5′-FR of CNR1 are both associated with HDL-C in vivo . These variants are tightly linked ( r 2 =0.925), and their minor alleles are commonly inherited together (as a diplotype, frequency ~15%). To determine their impact in EMSA, we first tested their collective impact on DNA binding using nuclear protein lysates from embryonic kidney cells (HEK293) ( Fig. 3a ). The presence of both rs806370 and rs806371 induced a super-shift band compared with combined major alleles when characterized by EMSA. Although our in vivo studies indicated that rs806370 and rs806371 are tightly linked, our in vitro studies indicate that only rs806371 introduces a novel DNA-binding site for nuclear proteins, based upon subsequent EMSA analyses conducted with probes for single variants ( Fig. 3a ). rs806371 decreases reporter gene expression To further characterize the functional role of rs806371 in the context of gene expression, and to quantify the direction of the effect, gene promoter reporter (luciferase) assays were conducted using site-directed mutagenesis. The CNR1 5′-FR (~3 kb immediately 5′ from the CNR1 transcription start site) was cloned upstream of Gaussian luciferase (secreted) in the the pEZX-PG04 reporter construct that also contains secretory alkaline phosphatase for transfection efficiency control analysis (see Methods). Owing to the observation that rs806371, not rs806370, was found to be the functional variant on EMSA, site-directed mutagenesis was used to create a representative rs806371 novel regulatory DNA binding site. After transfection into human hepatoma cells (Huh-7 cells), promoter reporter luciferase and control alkaline phosphatase activities were quantified serially in cultured media, over 3 days ( Fig. 3b ). Reporter gene expression, quantified by secreted luciferase activity, was markedly reduced by the presence of rs806371: ~25% reduction in activity at 48 h, and ~50% reduction at 72 and 96 h. There is growing evidence that genetic variation in CNR1 directly influences dysmetabolic traits in humans by altering the activity of CB 1 receptor-dependent signaling in peripheral tissues. We provide evidence in support of this claim through a novel series of experiments involving deep sequencing and comprehensive re-genotyping in a clinical practice-based biobank, followed by functional validation in two separate in vitro assay systems. Our results show that rs806371 in the CNR1 promoter alters HDL-C level in humans by generating a novel regulatory DNA-binding site capable of reducing CNR1 expression. Our current approach is unique. We had previously reported an association between CNR1 haplotype and circulating HDL-C levels in multi-generational families [13] . To narrow our search for the causal variant underlying this association, a 15-kb region of genomic DNA (containing the promoter, 5′-FR, coding region and 3′-UTR of the CNR1 gene) was sequenced, and all polymorphisms discovered in this region were re-genotyped in a biobank linked to EMRs [16] . In recent years, the use of EMRs has expanded rapidly (in response to the Affordable Care Act) creating huge longitudinal data sets ideal for observational research [20] , [21] , [22] , and BioVU at Vanderbilt University is currently the nation’s largest collection of DNA samples linked to EMRs ( n =157,719). Because of its unprecedented sample size and its unique design, we were able to leverage BioVU to identify a narrow region (~100 bp) within the CNR1 promoter associated with median HDL-C levels independent of BMI. The strength of this association did not change when our clinical practice-based lipid data were right-censored by exposure to lipid-modifying therapy (before censoring, mean HDL-C±s.d. was 53.47±16.45, 51.13±16.64 and 48.23±12.60 mg dl −1 for subjects with AA, AC and CC at rs806371; after censoring, mean HDL-C±s.d. was 52.71±16.80, 52.70±17.05 and 48.13±12.84 mg dl −1 for AA, AC and CC). In our primary analysis, two common variants within the 5′-FR, rs806370 and rs806371, were associated with median HDL-C level extracted from clinical data, after adjustment for BMI. As the effect size for each of these associations was clinically significant (~5 mg dl −1 change in HDL-C level) and nearly identical to the effect of our previously reported CNR1 risk haplotype ( Table 3 ), rs806370 and rs806371 were selected for further functional characterization in vitro . Even though these two SNPs are co-inherited, our data clearly indicate that rs806371, not rs806370, alters nuclear protein binding in an EMSA. As rs806371 markedly reduces reporter gene expression when engineered into a vector containing the CNR1 promoter, further studies are needed to define the transcription factors involved. Tissue-specific differences in transcription factors regulating the CNR1 locus (for example, within brain versus adipose tissue) may explain the fact that CB 1 receptor antagonists increase HDL-C, whereas CNR1 loss-of-function variants decrease HDL-C [23] . For example, insulin-dependent signaling in the brain engages different second messengers than peripheral tissues [24] , [25] . The degree to which these differences impact CNR1 expression remain uncharacterized. Physical interaction between our 5′ loss-of-function variant and CNR1 elements located more distally may also differ tissue by tissue. Within the current study, we also observed that HDL-C was associated with a rare variant located on the 3′-end of the gene. While this variant, CNR1-11675, was only observed in 2 of 1000 study subjects, the de-identified clinical data linked to these 2 samples revealed a marked elevation in HDL-C level (70.2±17.3 mg dl −1 , mean±s.d.) in the absence of an obvious clinical explanation for abnormal lipid homeostasis. Thus, additional work is needed to clarify the impact of these CNR1 variants on chromatin structure. Chromatin state predictions now available online for ENCODE indicate the presence of an insulator regulated by CTCF near CNR1 ( http://genome.ucsc.edu/cgi-bin/hgTracks?position=chr6:88847472-88881527&hgsid=325405609&wgEncodeUwHistoneViewHot=full ). Bioinformatic algorithms that predict transcription factor binding suggest additional regulatory mechanisms on the 5′-end; for example, the minor allele at rs806371 may disrupt a non-canonical glucocorticoid receptor (TRANSFAC V8.3 at http://alggen.lsi.upc.es/cgi-bin/promo_v3/promo/promo.cgi?dirDB=TF_8.3&calledBy=alggen ). Publically available eQTL data sets indicate that this locus also regulates the nearby RNGTT gene ( P =0.0273), in HapMap Europeans [23] . RNGTT is located just upstream of CNR1 (~400 kb), and it encodes an RNA guanylyltransferase recently associated with subcutaneous adipose tissue volume in women from the Framingham Offspring Study [26] . Clearly, the pathophysiological mechanism linking rs806371 to HDL-C level warrants further investigation. Endocannabinergic signaling alters HDL homeostasis through mechanisms that are both direct ( CNR1 expression in hepatocytes or adipocytes) [27] , [28] , [29] and indirect ( CNR1 expression in the brain) [30] . Non-brain-penetrant CB 1 receptor antagonists directly increase plasma HDL-C levels in animal models [31] , and CB 1 blockade modulates the release of adipocytokines from human adipocytes [29] , [30] , [32] , [33] . As these processes influence the intravascular remodeling of HDL particles in vivo [33] , [34] , [35] , CNR1 gene variability may influence public health by altering cardiovascular risk in the context of the current obesity epidemic [36] . Study population The current study was conducted in accordance with the Principles outlined within the Declaration of Helsinki. Approval was obtained from the Institutional Review Board of Vanderbilt University. The Vanderbilt DNA biobank (BioVU) currently contains EMRs from 157,719 subjects (updated 10 January 2013). BioVU accrues DNA samples extracted from blood drawn for routine clinical testing after these samples have been retained for 3 days and scheduled to be discarded. The DNA samples in BioVU are linked to a de-identified mirror image of each individual’s EMR. The current study cohort was randomly selected from ~100,000 unique individuals with European ancestry in BioVU. In order to reduce the potential data fragmentation caused by multiple health-care providers, we restricted study subjects to those listing Vanderbilt University Medical Center as their primary health care provider [37] , [38] . To do so, at least one note from general internal medicine was required. To enrich the data set for de-identified patient records containing dense longitudinal lipid data, at least three clinical lipid panels were also required for each subject. Using this approach, a total of 1,006 representative subjects were selected, including 509 females and 497 males. Phenotyping Outpatient median HDL-C levels represented our primary endpoint, available on all 1,006 subjects. Clinical lipid data were extracted from EMRs. These data reflected longitudinal lipid data (>10 years) collected during the course of routine clinical care. On average, each subject has 8 HDL-C values (ranging from 3–38 tests). All lipid data from inpatients were excluded as acute illness typically influences circulating lipid levels in most inpatients [39] . Data on lipid medications and related events (drug, dose, date and time) were also obtained from EMRs by applying our nature language processing algorithms [40] , [41] . Relevant clinical covariates were also obtained from EMRs. On average, each subject record had 18 glucose values (ranging from 1–196 tests) and 25 blood pressure values (ranging from 1–229 tests). Body mass index was calculated for each subject using median height and weight nearest the time stamp for median lipid values. When comparing our study cohort to the community of 1.8 million unique individuals from which this sample set was derived ( Table 1 ), no statistically significant difference was observed for BMI. However, there was a significant difference in median glucose levels ( P <0.001 additive model). As our inclusion criteria required dense longitudinal data (that is, at least three lipid panels per subject), our sampling process enriched for study subjects with regularly monitored cardiovascular risk factors. Thus, our sample was more likely to contain subjects with well-controlled diabetes mellitus. As anticipated, 250 of our 1,006 study subjects were diabetic, and because they were well-controlled, the mean glucose level in our overall sample was near normal (103.2±26.6 mg dl −1 , mean±s.d.) ( Table 1 ). Sequencing The CNR1 gene was completely sequenced in 95 individuals selected from Utah Centre d’Etude du Polymorphisme Humain (CEPH) HapMap reference panel (available from the Coriell Cell Repository, Camden, New Jersey, USA) [42] . A total of 15 kb genomic region was sequenced, including 5 kb upstream of the gene, 5 kb around the coding exon, and 5 kb downstream. Briefly, 5′-M13 tailed-gene-specific PCR primers were designed to cover the target region with amplicon sizes ranging from 500–750 bp with a minimum of 100 bp overlap between adjacent amplicons, where applicable, resulting in double-stranded coverage of all targeted regions. Overlapping amplicons were used to validate gene-specific primer sequences in independent experiments and rule out the possibility of allele-specific PCR amplifications. All primer sequences were compared with the whole-genome assembly to verify uniqueness against pseudogenes and gene families. Following temperature gradient optimization of small-scale reactions to determine optimal thermal cycling conditions, production-level PCR amplifications were performed in 96-well plates in a volume of 7 μl comprising 0.2 μl each of 7 μM forward and reverse primers, 2.8 μl DNA (5 ng μl −1 ), and 0.4 μl Elongase Enzyme (Invitrogen, Grand Island, New York, USA) or iProof polymerase (Bio-Rad, Hercules, California, USA) per well. Sequencing reactions were performed in MJ Tetrad PTC 225 thermal cyclers in 384-well format by using 5% BDT v3.1 sequencing chemistry (ABI, Foster City, California, USA). Chromatograms were generated from sequence reaction on an Applied Biosystems ABI 3730XL capillary sequencer. Data flow was tracked by using a custom-designed LIMS system at University of Washington. All chromatograms were base-called by using Phred, assembled into contigs by using Phrap, and scanned for SNPs with PolyPhred (v6.02) to identify polymorphic sites. Each chromatogram was trimmed to remove low-quality sequence (Phred score<25), resulting in analyzed reads averaging >450 bp with an average Phred quality of 40. Following assembly of all chromatograms onto an initial reference sequence, putative polymorphic sites were selectively reviewed by sequence analysts using Consed. Individual polymorphic sites in regions with lower quality data, ambiguous base calls, deviations from Hardy–Weinberg equilibrium (HWE) or those identified using laboratory quality control tools were reviewed to eliminate potential false-positive positions. Outlier genotypes (that is, deviations from HWE) were scrutinized by data analysts and removed from the data set if ambiguous. This approach generates sequence-based SNP genotypes with an accuracy of >99.9%. The results are publically available at Seattle SNPs on Genome Variation Server 134 at http://gvs.gs.washington.edu/GVS134/ . Genotyping Genotyping was performed on 1,006 DNA samples from BioVU using both common and rare variants identified from re-sequencing. As our sequencing efforts revealed no non-synonymous SNPs, three potential non-synonymous SNPs (rs78783387, rs75770301 and rs77016054) were included from existing databases. Two platforms were employed: six tagSNPs from our previous report [13] were genotyped using Taqman assay (ABI); all other polymorphisms were genotyped using iPLEX Gold assay (Sequenom, SanDiego, California, USA). MassARRAY Designer software was used to design iPLEX single base extension primers for multiplexed assays. Fifteen polymorphisms were rejected by the software and eliminated from genotyping. As a result, 54 polymorphisms were genotyped in the CNR1 genomic region on 1,006 subjects. All polymorphisms met a call-rate threshold of 94%. Except for rs806368 on the Taqman platform, all other SNPs had a call rate of >97%. Except for CNR1-4902 on the iPLEX Gold platform, all other SNPs had a call rate of >99%. Nine of these SNPs were monomorphic in BioVU, and they were removed from our analyses. All remaining SNPs followed H–W equilibrium. Electrophoretic mobility shift assays Double-stranded DNA probes (with or without rs806370 and rs806371) were prepared from biotin-labeled DNA oligos synthesized by IDT (Coralville, Iowa, USA). Nuclear protein was extracted with NE-PER nuclear extraction reagents (Pierce, Rockford, Illinois, USA), and each EMSA was performed with a Light Shift chemiluminescent EMSA kit (Pierce). For EMSA, the binding reactions were performed for 20 min in 1 × binding buffer, 5 mM MgCl2, 50 ng/μl poly(dI-dC), 0.05% Nonidet P-40, 2.5% glycerol, biotin-labeled probe, and nuclear protein extracts. Samples were electrophoresed on a native 6% polyacrylamide gel in 1 × Tris-borate-EDTA buffer and then transferred to a Biodyne membrane according to the manufacturer’s recommendation. For the competitive binding assay, non-labeled probes were added to the binding reaction at 200-fold excess over labeled probe [43] . Gene promoter reporter (luciferase) assays Approximately 3 kb of CNR1 5′-flanking region was amplified from human genomic DNA to create a reporter gene construct in pEZX-PG04 (GeneCopoeia, Rockville, Maryland, USA). Each genomic variant was introduced by circular PCR (QuikChange II XL Site-Directed Mutagenesis Kit, Agilent Technologies, Santa Clara, California, USA) and each insert was sequenced on both strands to avoid any amplification artifact or inadvertent inclusion of flanking polymorphisms. Constructs were transiently transfected into Huh-7 cells (500 ng). The assay was performed at 48, 72 or 96 h after transfection, and promoter reporter gene activity in cell lysates was measured using the Secrete-Pair Dual Luminescence Assay Kit (GeneCopoeia). Results were reported as the ratio of luciferase light units to secreted alkaline phosphatase, and the mean±s.e. has been illustrated in Fig. 3b . Statistics Each reporter gene assay was performed in triplicate. A student’s t -test was performed to evaluate the difference between groups. In BioVU, genotype–phenotype association tests were conducted using median lipid values as the primary endpoint, and all tests were performed using PLINK, a free, open-source genetic analysis toolset ( http://pngu.mgh.harvard.edu/~purcell/plink/ ). This platform was selected based on its efficiency, flexibility and ease of application. The --freq option was used to calculate minor allele frequency, and the --hardy option was used to calculate HWE. No SNPs in this study significantly deviated from HWE. A linear regression model was applied to test the relationship between each CNR1 variant and HDL-C level using the --linear option in PLINK. Asymptotic P -values were reported. An additive model, which fit our data best, was chosen for all analyses. We estimated the influence of covariates, including them in the linear regression model using the --covar option. We also reconstructed haplotypes using previously reported tag SNPs [13] . Haplotypes were estimated by applying standard E-M algorithms in the --hap option of PLINK. A linear regression model was applied to test each haplotype (versus all others), using the --hap-linear option. Only haplotypes with a frequency of ≥5% were included in these analyses. Accession codes: CNR1 SNP data have been deposited in Genbank under accession code KF042592 . How to cite this article: Feng, Q et al . A common functional promoter variant links CNR1 gene expression to HDL cholesterol level. Nat. Commun. 4:1973 doi: 10.1038/ncomms2973 (2013).